Genome-wide association study identifies peanut allergy-specific loci and evidence of epigenetic mediation in US children Food allergy (FA) affects 2%–10% of US children and is a growing clinical and public health problem. Here we conduct the first genome-wide association study of well-defined FA, including specific subtypes (peanut, milk and egg) in 2,759 US participants (1,315 children and 1,444 parents) from the Chicago Food Allergy Study, and identify peanut allergy (PA)-specific loci in the HLA-DR and -DQ gene region at 6p21.32, tagged by rs7192 ( P =5.5 × 10 −8 ) and rs9275596 ( P =6.8 × 10 −10 ), in 2,197 participants of European ancestry. We replicate these associations in an independent sample of European ancestry. These associations are further supported by meta-analyses across the discovery and replication samples. Both single-nucleotide polymorphisms (SNPs) are associated with differential DNA methylation levels at multiple CpG sites ( P <5 × 10 −8 ), and differential DNA methylation of the HLA-DQB1 and HLA-DRB1 genes partially mediate the identified SNP–PA associations. This study suggests that the HLA-DR and - DQ gene region probably poses significant genetic risk for PA. Food allergy (FA), defined as immunoglobulin E (IgE)-mediated clinical reactivity to specific food proteins, affects 2%–10% of children in the United States [1] , [2] . Over the past 20 years, FA has grown from a relatively uncommon to a major clinical and public health problem worldwide, due to its increasing prevalence, potential fatality and enormous medical and economic impact [3] , [4] , [5] . FA accounts for more than $20 billion in overall annual healthcare costs in the United States [5] . To date, there is no safe and effective prevention or treatment for FA, which is approved by the Food and Drug Administration for use in clinical practice, except for emergency management of allergic reactions induced by accidental exposure. Strict food avoidance is the only effective strategy to prevent future allergic reactions among FA patients; however, this is exceedingly difficult, as peanut, egg and cow’s milk (the three most common food allergens in the United States [3] ) are ubiquitous in processed foods. Indeed, a growing body of literature has shown that FA significantly diminishes quality of life among affected patients and their caregivers [3] , [6] , [7] , who live in constant fear of accidental ingestion and potentially life-threatening reactions. A major obstacle to effective prevention and treatment of FA is our limited understanding of its causes and underlying biological mechanisms. Although available data support a role for genetic factors in FA based on familial aggregation studies [8] , [9] and heritability estimates (ranging from 15% to 82%) [8] , [10] , few specific genes have been conclusively associated with FA, leaving its heritability largely unexplained. To date, all published genetic studies of FA have used a candidate gene approach, and have predominantly focused on peanut allergy (PA), a common type of FA that accounts for a disproportionate number of fatal and near-fatal food-induced episodes of anaphylaxis. Although multiple candidate genes have been reported for PA, few are considered established due to small sample sizes [11] , [12] , [13] , [14] , [15] , [16] , [17] , lack of adjustment for multiple comparisons [12] , [13] , [14] , [16] , [17] , [18] and a high failure rate in genotyping calls [18] . To our knowledge, loss-of-function mutations in the gene encoding filaggrin ( FLG ) are among the few genetic risk factors replicated for PA in multiple populations [19] , [20] , [21] . For other allergic diseases, genome-wide association studies (GWASs) have shown promise in recent years in dissecting the genetic basis of asthma [22] , [23] , [24] and atopic dermatitis [25] , [26] , [27] . Two recent GWASs have examined allergen sensitization [28] and self-reported environmental allergy [29] . These previous GWASs did not specifically examine FA, but did reveal substantial differences in genetic effects across various allergies [29] . Clinical FA is distinct from sensitization to foods or aeroallergens: a sensitized child may or may not manifest clinical signs or symptoms of FA, underscoring the need to explore genetic variants specifically associated with clinical FA (a growing clinical and public health challenge). Epigenetic mechanisms by which genetic variants affect FA are largely unexplored. DNA methylation (DNAm), a type of epigenetic mark, regulates gene expression. There is growing evidence that genetic variants can affect DNAm [30] , [31] , and that DNAm may mediate genetic susceptibility to autoimmune disease [32] . To date, no published study on FA has simultaneously considered genome-wide genetic and epigenetic factors, nor have they assessed whether DNAm could mediate genetic susceptibility to FA. To our knowledge, this is the first GWAS of well-defined FA in a US cohort of children and their biological parents. This study comprises three stages. In stage I, we use the modified quasi-likelihood score (MQLS) test [33] , [34] to detect genetic associations with any FA (including nine foods as follows: peanut, egg white, cow’s milk, soy, wheat, walnut, fish, shellfish and sesame seed) and the three most common types of FA (peanut, egg white and cow’s milk). We identify PA-specific loci in the human leukocyte antigen ( HLA)-DQ and -DR region at 6p21.32, tagged by rs7192 and rs9275596, respectively. In stage II, we perform a replication study of identified single-nucleotide polymorphisms (SNPs) from stage I in an independent sample from the same cohort, and confirm that both rs7192 and rs9275596 are significantly associated with PA. In stage III, we examine relationships between the two PA-associated SNPs and DNAm, between genotype-dependent DNAm and PA, and also whether DNAm mediates identified SNP–PA associations. We find that both SNPs are significantly associated with differential DNAm at multiple CpG sites and differential DNAm of the HLA-DQB1 and HLA-DRB1 genes partially mediate the identified SNP–PA association. The population attributable risk (PAR) is 21% and 19%, respectively, for rs7192 and rs9275596. Taken together, this study indicates the possibility that the HLA-DR and -DQ gene region likely poses the single greatest genetic risk for PA. Phenotype definition and population characteristics This study includes three stages as shown in Fig. 1 . Both discovery and replication samples were from the Chicago Food Allergy Study and were collected under a standard study protocol, as described in the Methods. Main phenotypes of interest included ‘any FA’ and the three most common types of FA: PA, egg allergy and milk allergy. As described in our previous report [35] , we applied stringent clinical criteria to define specific types of FA as follows: (1) a convincing history of clinical allergic reaction on ingestion of a specified food and (2) evidence of sensitization to the same food, defined as having a detectable food-specific IgE (≥0.10 kU l −1 ) and/or a positive skin prick test (SPT) with mean weal diameter (MWD)≥3 mm to this specified food (see Methods). Accordingly, we defined specific types of FA to nine common foods (accounting for >95% of all FAs in the population) and defined a child as having any FA if she/he was allergic to any of the nine foods. In the genetic association analyses, we also performed sensitivity analysis using other cutoffs for food-specific IgE and SPT to define FA, for example, food-specific IgE≥0.35 kU l −1 , SPT MWD≥5 mm (ref. 36 ) or either food-specific IgE or SPT MWD ≥95% positive predictive value (PPV). 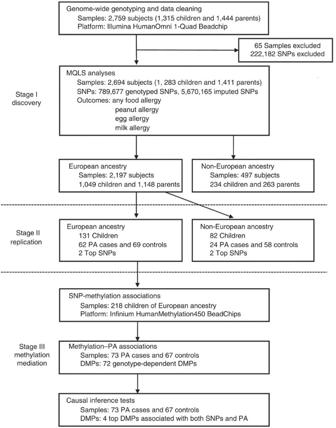Figure 1: Study design and work flow diagram for the GWAS of FA. DMP, differentially methylated position; MQLS, modified quasi-likelihood score analyses; PA, peanut allergy; SNP, single-nucleotide polymorphism. Figure 1: Study design and work flow diagram for the GWAS of FA. DMP, differentially methylated position; MQLS, modified quasi-likelihood score analyses; PA, peanut allergy; SNP, single-nucleotide polymorphism. Full size image GWAS to identify susceptibility loci for FA (Stage I) A total of 2,759 samples (1,315 children and 1,444 biological parents) from the Chicago Food Allergy Study [9] , [35] were genotyped using the Illumina HumanOmni1-Quad BeadChip. We performed vigorous quality control and thorough data cleaning as detailed in Methods. The final sample size for gene discovery (Stage I) included 2,197 individuals of European ancestry (671 FA-affected children) and 497 individuals of non-European ancestry (155 FA-affected children). Each individual’s genetic ancestry was estimated by principal component analysis (PCA) [37] by using the 1000 Genomes Project as a reference. The demographic and clinical characteristics of all study participants are provided in Supplementary Table 1 . The Stage I analyses included primarily family-based samples, with a small number of case–control samples. The MQLS test [33] , [34] was applied to test for genetic associations with FA due to its capacity to maximally use available information contained in the complex family data set (see Methods). The MQLS test allows for two types of controls: unaffected controls and controls of uncertain phenotypes. In this study, the children who did not meet FA case or control definitions and all parents were coded as controls of uncertain phenotypes (see Methods). We also performed sensitivity tests in different ways to incorporate controls of uncertain phenotypes. To minimize population stratification, we first performed the MQLS test in 2,197 individuals of European ancestry, and then examined whether the identified genome-wide significant association signals were also present in 497 individuals of non-European ancestry. The quantile–quantile plots for association analyses in 2,197 individuals of European ancestry indicated no inflation of the MQLS test due to cryptic population structure or unaccounted relatedness among individuals ( Fig. 2 and Supplementary Fig. 1 ). 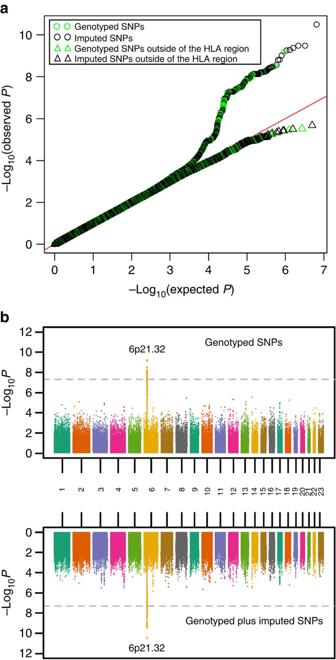Figure 2: Quantile–quantile (Q–Q) and Manhattan plots for genome-wide associations of PA in 2,197 discovery samples of European ancestry. (a) Q–Q plots for all of the genotyped and/or imputed SNPs and SNPs outside of the HLA-DQ and -DR region. (b) Manhattan plots for the genotyped SNPs alone (upper panel) and for the genotyped plus imputed SNPs. SNPs above the dashed line reached genome-wide significance at 5 × 10−8, based on the MQLS test. Figure 2: Quantile–quantile (Q–Q) and Manhattan plots for genome-wide associations of PA in 2,197 discovery samples of European ancestry. ( a ) Q–Q plots for all of the genotyped and/or imputed SNPs and SNPs outside of the HLA-DQ and -DR region. ( b ) Manhattan plots for the genotyped SNPs alone (upper panel) and for the genotyped plus imputed SNPs. SNPs above the dashed line reached genome-wide significance at 5 × 10 −8 , based on the MQLS test. Full size image We performed the MQLS test to examine genome-wide associations for any FA in 2,197 individuals of European ancestry, including 671 FA cases, 144 non-allergic non-sensitized normal controls and 1,382 controls of uncertain phenotypes (234 children and 1,148 parents). Under an additive model for the minor allele of each SNP, we found that no SNP reached genome-wide significance ( P <5 × 10 −8 ) or suggestive ( P <1 × 10 −7 ) threshold ( Table 1 ). Removing the 234 children with uncertain phenotypes from these analyses did not substantially change the results. Table 1 The top loci associated with FA and the three most common types of FA in 2,197 discovery samples of European ancestry. Full size table We further examined genome-wide associations for PA, egg allergy and milk allergy among 2,197 individuals of European ancestry. In 316 PA cases, 144 non-allergic non-sensitized controls and 1,737 controls of uncertain phenotypes (589 children and 1,148 parents), the MQLS test identified genome-wide significant associations for 40 SNPs spanning the HLA class II DQ genes at the 6p21.32 region ( Fig. 2 and Supplementary Table 2 ). An intergenic SNP, rs9275596, between the HLA-DQB1 and HLA-DQA2 genes, showed the most significant association with PA ( P =6.8 × 10 −10 ; Fig. 3 and Supplementary Table 2 ). The other 39 SNPs were predominantly in moderate-to-strong linkage disequilibrium (LD) with rs9275596 ( Fig. 3 and Supplementary Table 2 ), and their associations with PA were no longer significant when conditioning on rs9275596 (all P >0.001), suggesting that this group of SNPs represents a single significant genetic signal for PA. At >200 kb upstream from this significant signal, eight SNPs located within or clustered around the HLA-DRA gene were in strong LD with each other ( r 2 =1) and showed suggestive associations with PA ( P <1 × 10 −7 ; Fig. 3 ). Among these identified SNPs, rs7192 ( P =5.5 × 10 −8 ) was the only coding SNP that leads to a Leu242Val change in the HLA-DRA gene product. The odds ratio (OR) and 95% confidence intervals (CIs) were the same for one copy of the rs7192-T allele and one copy of the rs9275596-C allele: 1.7 (95% CI: 1.4–2.1), as estimated by a generalized estimating equation (GEE) regression model ( Table 2 ). The association between rs9275596 and PA was significantly reduced (OR=1.4, 95% CI=1.1–1.8, P =0.01) when conditioned on rs7192, suggesting that SNP rs9275596 and rs7192 may represent a single risk factor for PA. 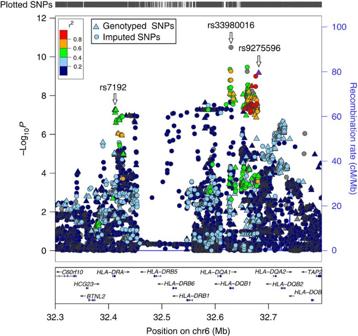Figure 3: Locus-specific plot of PA-associated loci reaching genome-wide significance. Each dot represents the −log10(P-value) for one genotyped or imputed SNP based on the MQLS test in 2,197 discovery samples of European ancestry. The estimated recombination rates from the 1000 Genomes Project data are shown as blue lines and the genomic locations of genes within the regions of interest are shown at the bottom. SNP colour represents LD with the most significant genotyped SNP (rs9275596). SNP annotations are indicated as follows: triangles, genotyped SNPs; circles, imputed SNPs. Figure 3: Locus-specific plot of PA-associated loci reaching genome-wide significance. Each dot represents the −log 10 ( P -value) for one genotyped or imputed SNP based on the MQLS test in 2,197 discovery samples of European ancestry. The estimated recombination rates from the 1000 Genomes Project data are shown as blue lines and the genomic locations of genes within the regions of interest are shown at the bottom. SNP colour represents LD with the most significant genotyped SNP (rs9275596). SNP annotations are indicated as follows: triangles, genotyped SNPs; circles, imputed SNPs. Full size image Table 2 The estimated effect sizes of the two top SNPs on risk of PA in the discovery and replication samples. Full size table We performed a sensitivity test to examine whether the identified genetic associations for PA varied by IgE or SPT cutoffs. As shown in Table 3 , the estimated ORs for either rs7192 or rs9275596 remained similar when more stringent IgE or SPT cutoffs were applied. We then tested associations for rs7192 and rs9275596 with PA, in 497 individuals of non-European ancestry. No significant associations were detected ( Table 2 ). These results were unchanged when a quantitative version of MQLS analyses was applied to adjust for ancestry based on the first three principal components (PCs) from the genome-wide SNP genotypes. Table 3 Associations of the two top SNPs with PA based on various definitions in 2,197 discovery samples of European ancestry. Full size table The MQLS test for egg allergy and milk allergy did not identify any genome-wide significant or suggestive SNPs in the 2,197 individuals of European ancestry, and the two PA-associated SNPs (rs7192 and rs9275596) showed no evidence of association with either egg or milk allergy ( Table 1 ). Neither rs7192 nor rs9275596 showed associations with other allergic phenotypes in 2,197 individuals of European ancestry ( Supplementary Table 3 ). SNP imputation was also conducted in this study. With the latest versions of SHAPEIT [38] and IMPUTE2 (ref. 39 ), a total of 6,459,842 genotyped and/or imputed SNPs passed post-imputation quality control steps (see Methods) and were then tested for their associations with each outcome (any FA, PA, egg allergy and milk allergy) among 2,197 individuals of European ancestry. The MQLS test for PA revealed a single genome-wide significant peak at 6p21.32, the same region identified in our original analysis of genotyped SNPs alone ( Fig. 2 ), but the peak now included an additional 99 imputed SNPs ( Supplementary Table 2 ). Imputed SNP rs33980016 (an insertion/deletion SNP in the intronic region of the HLA-DQB1 gene) showed the most significant association with PA ( P =3.2 × 10 −11 ; Fig. 3 ); it was in moderate LD ( r 2 =0.54) with genotyped SNP rs9275596. When conditioned on the genotyped SNP (rs9275596 or rs7192), the association between rs33980016 and PA was largely reduced ( P >0.001), suggesting that these imputed and genotyped SNPs may represent one single genetic region. No genome-wide significant or suggestive associations were identified for any FA and egg allergy ( Supplementary Fig. 1 ). Four imputed SNPs on chromosome 3, located between the C3orf67 and LOC339902 genes, showed suggestive associations ( P <5 × 10 −7 ) with milk allergy. However, this suggestive peak appears to be driven by imputed SNPs, because there is no such association based on genotyped SNPs in this region ( Supplementary Fig. 1 ). As no genome-wide significant associations were found for any FA, egg allergy or milk allergy, we narrowed the scope of our replication and DNAm mediation analyses to focus on PA. Replication and meta analyses (Stage II) We performed a replication study for two genotyped PA-associated SNPs, rs9275596 (the most significant genotyped SNP for PA) and rs7192 (a potential functional SNP), in an independent sample (86 PA cases and 127 controls) from the same Chicago Food Allergy cohort. Sample selection criteria and data cleaning procedures are provided in Methods. 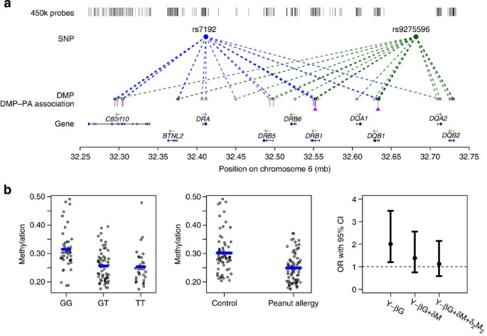Figure 4: DMPs associated with rs7192, rs9275596 and with PA, as well as DMPs that mediate genetic risk in PA. (a) Diagram showing associations between genotype (rs7192 (blue circle) and rs9275596 (green circle)) and DMPs, and between the genotype-dependent DMPs and PA. The DMPs are denoted by empty circles. Dashed blue (for rs7192) and green (for rs9275596) lines represent significant associations between genotypes and DMPs atP<5 × 10−8based on linear regression models (N=218). In between the DMPs and gene tracks are purple bars that represent the genotype-dependent DMPs that are associated with PA based on linear regression models in 73 PA cases and 67 non-PA controls (DMPs as the outcomes). The two DMPs marked with purple triangles are DMP cg15982117 in theHLA-DRB1gene and DMP cg18024368 in theHLA-DQB1gene that may mediate genetic risk in PA, as determined by the CIT. (b) DMP cg18024368 in theHLA-DQB1gene that may mediate the association between the rs7192 genotype and PA risk in 73 PA cases and 67 non-PA controls. The left panel shows the association between the methylation level at DMP cg18024368 and the rs7192 genotype. The middle panel depicts the association between the methylation level at DMP cg18024368 and PA. The blue bars in the left and middle panels represent median methylation levels. The right panel shows the effect size of the observed rs7192–PA associations (represented by ORs based on the logistic regression model) before and after adjusting for the methylation level at DMP cg18024368 (M), as well as adjusting for both the methylation level at DMP cg18024368 (M) and at DMP cg15982117 (M2). Error bars represent the 95% CIs of the estimated ORs. The demographic characteristics of the replication sample are presented in Supplementary Table 4 . There were 131 children (62 PA cases and 69 controls) of European ancestry and 82 of non-European ancestry (24 PA cases and 58 controls) based on PCA analysis. Using GEE models to account for correlations among the 23 sibling pairs and to adjust for age and gender, we found that both rs7192 (OR=1.8, 95% CI=1.2–2.7, P =0.005) and rs9275596 (OR=1.7, 95% CI=1.1–2.6, P =0. 022) were significantly associated with PA after Bonferroni correction ( P <0.025 for two SNP tests) in children of European ancestry, and that both SNPs had a similar effect size as seen in the Stage I GWAS results ( Table 2 ). No such associations were detected in children of non-European ancestry ( Table 2 ). Using allele frequencies reported in the HapMap Utah Residents with Northern and Western European Ancestry (CEU) and ORs derived from the replication sample of European ancestry (to avoid ‘winner’s curse’ bias), we estimated the PAR, which was 21% for rs7192 and 19% for rs9275596. DNAm mediation (Stage III) In 218 unrelated children of European ancestry (including 73 PA cases, 67 non-PA controls and 78 children with uncertain PA phenotype), we tested associations between the top genotyped SNPs (rs7192 and rs9275596) and whole-blood DNAm levels at genome-wide CpG sites derived from the Infinium HumanMethylation450 BeadChip. When adjusting for age, gender and estimated cell composition (see Methods), we identified 72 differentially methylated positions (DMPs, P <5 × 10 −8 ): 69 located at chromosome 6p21.32 ( Fig. 4a ), 1 at 7q22 (cg03324851 in the GNB2 gene), 1 at 12q24.33 (cg01256320 in the FBRSL1 gene) and 1 at 17q25.1 (cg12311094 in the C17orf77 gene). Of these 72 DMPs, 29 were significantly associated with rs7192 and rs9275596 (the top PA-associated genotyped SNPs), 17 were significantly associated with rs7192 and the remaining 26 DMPs were significantly associated with rs9275596. Figure 4: DMPs associated with rs7192, rs9275596 and with PA, as well as DMPs that mediate genetic risk in PA. ( a ) Diagram showing associations between genotype (rs7192 (blue circle) and rs9275596 (green circle)) and DMPs, and between the genotype-dependent DMPs and PA. The DMPs are denoted by empty circles. Dashed blue (for rs7192) and green (for rs9275596) lines represent significant associations between genotypes and DMPs at P <5 × 10 −8 based on linear regression models ( N =218). In between the DMPs and gene tracks are purple bars that represent the genotype-dependent DMPs that are associated with PA based on linear regression models in 73 PA cases and 67 non-PA controls (DMPs as the outcomes). The two DMPs marked with purple triangles are DMP cg15982117 in the HLA-DRB1 gene and DMP cg18024368 in the HLA-DQB1 gene that may mediate genetic risk in PA, as determined by the CIT. ( b ) DMP cg18024368 in the HLA-DQB1 gene that may mediate the association between the rs7192 genotype and PA risk in 73 PA cases and 67 non-PA controls. The left panel shows the association between the methylation level at DMP cg18024368 and the rs7192 genotype. The middle panel depicts the association between the methylation level at DMP cg18024368 and PA. The blue bars in the left and middle panels represent median methylation levels. The right panel shows the effect size of the observed rs7192–PA associations (represented by ORs based on the logistic regression model) before and after adjusting for the methylation level at DMP cg18024368 ( M ), as well as adjusting for both the methylation level at DMP cg18024368 ( M ) and at DMP cg15982117 ( M2 ). Error bars represent the 95% CIs of the estimated ORs. Full size image The 72 identified genotype-dependent DMPs were then tested for their associations with PA in 73 PA cases and in 67 non-PA controls. The estimated proportion of CD4T cells in whole blood was slightly lower in PA cases than in controls ( P =0.02). With the adjustment for age, gender and estimated cell composition, a total of 18 DMPs, located in the c6orf10 ( N =7), HLA-DRB5 ( N =2), HLA-DRB1 ( N =8) and HLA-DQB1 ( N =1) genes, respectively, were significantly associated with the risk of PA after Bonferroni correction ( P <0.0005) and showed a ≥5% adjusted methylation level difference between PA cases and controls ( Fig. 4a ). For each of the four identified genes ( c6orf10 , HLA-DRB5 , HLA-DRB1 and HLA-DQB1 ), the top DMP, which was (1) significantly associated with both rs7192 and rs9275596 ( P <5 × 10 −8 ), and (2) yielded the smallest P- value in association tests with PA, was further tested for its role in mediating the SNP–PA association via a causal inference test (CIT) ( Table 4 ). Briefly, to be a qualified mediator, this CIT must meet the following criteria [32] , [40] : (i) genotype and PA are associated; (ii) genotype is associated with DMP independent of PA; (iii) DMP is associated with PA independent of genotype; and (iv) genotype is not independently associated with PA after adjusting for DMP. We found cg15982117 in the HLA-DRB1 gene and cg18024368 in the HLA-DQB1 gene significantly mediated the effects of rs7192 and rs9275596 on PA ( Table 4 , all P CIT <0.005) after Bonferroni correction for four different DMPs and two different SNPs. As an example, Fig. 4b shows that DMP cg18024368 in the HLA-DQB1 gene was significantly hypomethylated in children carrying the T risk allele at rs7192 ( P =2.7 × 10 −10 ; Fig. 4b , left panel) and also in PA cases ( N =73) compared with non-PA controls ( N =67, P =2.4 × 10 −6 ; Fig. 4b , middle panel). The estimated OR for the rs7192–PA association was substantially reduced after adjusting for DMP cg18024368, suggesting that this DMP acts as a mediator ( P CIT= 0.002, Bonferroni adjusted P CIT =0.016; Table 4 ). Similar associations were found for DMP cg15982117 in the HLA-DRB1 gene ( Table 4 and Supplementary Fig. 3 ), and the estimated OR for the rs7192–PA association was close to 1.0 after adjusting for both DMPs (cg18024368 and cg15982117; Fig. 4b , right panel). Table 4 Differentially methylated positions that mediate genetic risk in PA. Full size table Additional supporting analyses To maximize the study power, we performed genome-wide meta-analysis for PA across the discovery and the replication samples of European ancestry (total N =2,328) using 5,693,167 imputed and genotyped autosomal SNPs (see Methods). Imputed SNP rs33980016 in the HLA-DQB1 gene remained the top SNP for PA ( P meta =2.9 × 10 −12 ), followed by imputed SNP rs9273841 ( P meta =5.2 × 10 −11 ) and genotyped SNP rs9275596 ( P meta =6.3 × 10 −11 ; Supplementary Table 2 and Supplementary Fig. 2 ). SNP rs7192 was also significantly associated with PA ( P meta =2.8 × 10 −9 ) ( Table 2 ). These findings further support that the 6p21.32 region is significantly associated with the risk of PA. No additional significant/suggestive signals outside of the 6p21.32 region were identified. Given the unique LD pattern in the HLA region, we imputed the classical HLA alleles in individuals of European ancestry using the HLA*IMP framework [41] . In the discovery stage, 50 HLA alleles in the major histocompatibility complex ( MHC ) class II region with a frequency of 0.02 or above were analysed for possible association with PA. HLA-DQA1*0102 was the only risk allele significantly associated with PA ( P =4.5 × 10 −8 ). This was confirmed in the replication sample of European ancestry ( P =0.025) and in meta-analysis ( P meta =5.0 × 10 −9 ; Supplementary Table 5 ). To compare the relative effects of different HLA variants in association with PA, we imputed classical two-digit and four-digit HLA alleles, and amino acid (AA) polymorphisms in the MHC class II region, using the SNP2HLA framework [42] . The four-digit classical HLA alleles imputed by SNP2HLA were concordant with those imputed by HLA*IMP and HLA-DQA1 *0102 continued to be significantly associated with PA. A two-digit classical HLA allele, HLA-DQB1*06 , was also significantly associated with PA in both the discovery and the replication samples of European ancestry ( Supplementary Table 5 ). Similar associations were found for these two genes when AA polymorphisms were analysed instead ( Supplementary Table 5 ). Among all of the classical HLA alleles and AA polymorphisms tested, the AA polymorphism at position 71 in the HLA-DRB1 gene showed the top association signal with PA in both the discovery stage ( P =2.3 × 10 −10 ) and in the meta-analysis ( P meta =9.8 × 10 −11 ), in which the presence of Arg at position 71 was associated with a decreased risk of PA ( Supplementary Table 5 ). A similar association trend was also found for this polymorphism in the replication sample, although it was statistically insignificant ( P =0.189). All of these associations were greatly reduced by conditioning on rs9275596 or rs7192 ( P >0.008), suggesting that these identified classical HLA alleles and/or AA polymorphisms may not be independent of the two validated PA-associated SNPs reported here. By querying existing expression quantitative trait loci (eQTL) databases for populations of European ancestry, we found both rs7192 and rs9275596 were significantly associated with expression levels of the HLA-DRA , HLA-DRB5 , HLA-DRB1 , HLA-DQA1 , HLA-DQB1 and HLA-DQA2 genes in subcutaneous/omental adipose [43] , liver [43] and lymphoblastoid cell lines ( http://regulome.stanford.edu ; Supplementary Table 6 ) [44] , [45] , [46] . We then explored the most significant cis -eQTLs for these six genes in subcutaneous/omental adipose and liver cell lines, separately ( Supplementary Table 7 ). SNP rs7192 was in almost complete LD ( r 2 =0.99) with rs3763327 (an intergenic SNP between the HLA-DRA and HLA-DQB9 genes), the most significant cis -eQTL of the HLA-DRA gene in the liver, and the association between rs7192 and HLA-DRA1 gene expression ( P =1.9 × 10 −16 ) was comparable to that of rs3763327( P =1.8 × 10 −16 ). These results indicate that rs7192 is a potential cis -QTL of the HLA-DQA1 gene in the liver ( Supplementary Table 7 ). In contrast, rs9275596 was in low-to-moderate LD ( r 2 <0.61) with the most significant eQTL for each gene–tissue combination. There is growing evidence that genetic factors may play a role in FA; however, there is a particular lack of knowledge regarding the genetic and epigenetic underpinnings of FA as a whole and also its subtypes [47] . We conducted the first GWAS study of well-defined FA, including specific subtypes (peanut, milk and egg) in US children, a particularly important age group given that FA most commonly develops in early childhood. In addition, this is the first study to demonstrate the key role of differential DNAm in mediating identified genetic risk factors for PA. Specifically, we identified and replicated genetic variants in the HLA-DR and -DQ gene region that were significantly associated with PA in children of European ancestry, tagged by rs7192 (a non-synonymous SNP of the HLA-DRA gene) and/or rs9275596 (intergenic between the HLA-DQB1 and HLA-DQA2 genes). Both rs7192 and rs9275596 significantly affect DNAm in several nearby genes. DNAm in the HLA-DRB1 and HLA-DQB1 genes, in turn, mediate the detected SNP–PA associations. Taken together with a PAR of 19%–21%, this GWAS indicates the possibility that the HLA-DR and -DQ gene region likely poses the single greatest genetic risk for PA. The role of HLA variants in PA has been examined by previous candidate gene studies via direct assessment of HLA classical alleles [12] , [13] , [14] , [16] , [17] , [18] , but the results were inconclusive, partly due to relatively small sample sizes and inadequate control of potential population stratification. This GWAS provides convincing evidence that the HLA-DR and -DQ gene region, as tagged by rs7192 or rs9275596, harbours significant genetic risk for PA in subjects of European ancestry. These two SNPs may represent one single risk factor, as the association between rs9275596 and PA was not independent of rs7192. To maximize the study power, we conducted a meta-GWAS across the discovery and the replication samples on a combined set of genotyped and imputed SNPs, which further supports this HLA-DR and -DQ gene region as a single significant region for PA. Our findings are biologically plausible. The HLA-DR and -DQ molecules, which are expressed in a range of cells, including B cells, activated T cells and the monocyte/macrophage lineage, are known to play a critical role in the development of allergy [48] . These molecules present antigen-derived peptides, mostly of exogenous origin, to CD4+ helper T cells. Antigen presentation by HLA molecules is a defining step in the development of antigen-specific immune responses. These molecules have extensive molecular polymorphisms confined to the peptide-binding groove. These polymorphisms may determine which antigen-derived peptides are bound and presented to T cells via T-cell receptors, and may account for allergen-specific sensitivities. The top PA-associated AA polymorphism, at position 71 in the HLA-DRB1 gene (imputed by SNP2HLA), is one such polymorphism located in the peptide-binding groove and may partly account for the identified associations. Previous studies have shown that this AA position, together with positions 13, 70 and 74, play important roles in the binding-specificity profile of pocket 4, which is one of the most important pockets for antigen interaction and presentation by the HLA-DR molecule [49] . Another possible explanation for our findings is that rs7192, a missense SNP in the HLA-DRA gene, may directly affect HLA-DRA protein function and/or expression and thus affect binding of HLA molecules with peanut allergens. This SNP was significantly associated with HLA-DRA gene expression in multiple tissues including adipose, liver and lymphoblastoid cell lines, which probably represent associations in antigen presenting cells throughout the body. In the liver, rs7192 may be an actual eQTL of the HLA-DRA gene, because (1) it is in almost complete LD with the top cis -eQTL (rs3763327) of the HLA-DRA gene ( r 2 =0.99) and (2) it induces a Leu242Val change in the HLA-DRA gene, while rs3763327 is an intergenic SNP between the HLA-DRA and HLA-DQB9 genes with unknown functionality. The liver has been demonstrated to play a critical role in oral tolerance induction [50] . It would be of great interest to further examine these associations in additional tissues such as the intestinal mucosa and skin, which are likely to be critical to the pathogenesis of PA. We still cannot exclude the possibility that other untyped variants that are in high LD with rs7192 or rs9275596 could be the causal SNP(s). Although the imputed SNP, rs33980016, showed the strongest association with PA, our conditional analyses indicate that this top SNP signal is not distinguishable from the signals at rs9275596 or rs7192 with our current data. Our data provide strong evidence that the 6p21.32 region poses significant risk for PA. However, targeted sequencing in this region is needed to more precisely identify and validate the causal variant(s) for PA. There is growing evidence that genotype may control DNAm levels [30] , [31] . DNAm, which regulates gene expression, might influence disease development in a manner complementary to direct mutation of the DNA sequence itself. A recent small epigenome-wide association study identified DMPs in the HLA-DQB1 gene for IgE-mediated FA [51] . Genetic and epigenetic modification may also interact biologically [52] . We showed that both rs7192 and rs9275596 were methylation quantitative loci for the HLA-DRB1 and HLA-DQB1 genes, and that there are significant causal relationships among the genotypes, DNAm and the risk of PA. This indicates that DNAm may regulate the expression levels of these genes and, subsequently, may partly mediate the genetic risk of PA. A similar linkage was observed for rheumatoid arthritis in a recent study, although the involved SNPs and DMPs in the HLA region were not the same as those identified in our study [32] . Given the genetic associations with the HLA region and disease pathogenesis that have already been linked to specific HLA protein epitopes, the methylation mediation observed here implies an additional complementary mechanism by which the HLA variants may influence PA. This study represents the first step in understanding the role of DNAm mediation effects on PA. Our findings provide clues and underscore the need for additional functional studies, including follow-up data on independent PA subjects in a clinical setting, to show how genotype-dependent DNAm could regulate the expression of key genes, and how these expression patterns may correlate with clinical outcomes. Longitudinal cohort studies on DNAm at multiple time points are also needed to assess dynamic changes in DNAm and its temporal relationship with the risk of PA. We showed that the identified SNP–PA associations were not observed for milk allergy, egg allergy or other allergic phenotypes (including allergic sensitization, self-reported physician-diagnosed asthma, eczema and allergic rhinitis; Supplementary Table 3 ), raising the possibility that PA may be under distinct genetic control. However, this study is underpowered on a genome-wide level, both for ‘any FA’ and for its subtypes. The finding of an association with PA should be interpreted cautiously in the context of limited study power. The lack of association between the two PA-associated SNPs, and other FA and/or other allergic phenotypes may be due to limited sample size and limited study power, hence requiring further studies in a larger sample. Our study is also limited in the following aspects. As is the case in most GWAS studies, we examined the genetic associations for common variants. Substantially larger sample sizes will be required to identify rare variants or common variants with small effects. We replicated our GWAS results in an independent set of samples from the same Chicago Food Allergy Study. Our findings could be further strengthened by additional replications in other independent populations. The significant associations that we identified between rs7192 and rs9275596 and PA were not present in the participants of non-European ancestry; however, we cannot firmly conclude that these effects are specific to population of European ancestry due to a limited sample size of non-Europeans. Batch effect is one of the major problems often encountered in epigenetic studies [53] . We used ComBat [54] transformation of methylation data to minimize potential confounding by batch effects. After transformation, the average DNAm level of the reported DMPs in PA cases or controls did not vary significantly across plates. Another issue linked to epigenetic studies is related to tissue- and cell-specific characteristics. FA is a systemic condition for which the study of methylation patterns in blood may be feasible, although cell heterogeneity in blood may act as a potential confounder [55] , [56] due to the cell-specific pattern of DNAm [57] . Accordingly, we adjusted for estimated cell composition using the ‘limma’ package [58] in all epigenetic association tests. However, we could not exclude the possibility of some residual confounding. The identified DNAm mediation effects will require replication and verification in future studies. In summary, this GWAS of FA revealed one significant peak at 6p21.32 for PA, and the finding appears to be consistent based on analyses of genotyped SNPs, imputed SNPs, imputed classical HLA alleles and AA polymorphisms, and a meta-GWAS across the discovery and replication samples. Specifically, this study identified PA-specific susceptibility loci in the HLA-DQ and -DR region at 6p21.32, tagged by rs7192 and rs9275596. Both SNPs were associated with differential DNAm levels at multiple CpG sites and differential DNAm of the HLA-DQB1 and HLA-DRB1 genes partially mediated the identified SNP–PA association. Taken together with a PAR of 19%–21%, this study indicates the possibility that the HLA-DR and -DQ gene region likely poses the single greatest genetic risk for PA. Findings from this study warrant additional replication, validation and functional studies, which will have the potential to improve our understanding of the genetic factors and epigenetic mechanism underlying the risk of PA, and may inform future development of new strategies for the prediction, prevention and treatment of PA. The Chicago Food Allergy Study Both the discovery and replication samples were enrolled as part of the Chicago Food Allergy Study under a standard study protocol. All participants were recruited from the Chicago area from August 2005 to June 2011. Eligible families were those having either one or both parents with at least one biological child (aged 0–21 years) with or without FA, willing to participate in the study. Eligible FA case or control children (aged 0–21 years) were those with or without FA. For each family or participant, the following procedures were completed: (1) questionnaire interview by trained research staff to obtain information on each family member’s home environment, diet, lifestyle, history of FA and other allergic diseases; (2) clinical evaluation by nurse or trained research staff to obtain height, weight, waist and hip circumference, blood pressure measurement and lung function test; (3) allergy SPT; and (4) collection of venous blood samples for food specific IgE (sIgE) measurement, DNA extraction and subsequent laboratory assays. Detailed information on SPT and sIgE measurement is given in the Supplementary Methods . For each child, we also collected a detailed history of clinical allergic reaction on ingestion of specific foods. The study protocol was approved by the Institutional Review Board of Ann and Robert H. Lurie Children’s Hospital of Chicago and the Institutional Review Board of Johns Hopkins Bloomberg School of Public Health. Written informed consents were obtained from all participants or their legal guardian (for children aged <18 years). Study sample included in the current GWAS of FA In the discovery stage, we primarily used samples from nuclear families. A total of 2,759 subjects (853 families) were included. Among these families, 780 families ( n =2,678) were included based on the following criteria: (1) at least one child had a convincing history of clinical allergic reaction on ingestion of specific foods and (2) two or more additional family members (parents/siblings) had archived DNA samples. Another 81 children from 73 families without parental genotyping data were also included (29 FA cases and 52 controls). In the replication stage, we aimed to replicate the identified genetic associations with PA. We included 216 case–control samples (88 PA cases and 128 controls) from the Chicago Food Allergy Study, all independent of the discovery sample. Definitions of phenotypes of interest The main phenotypes of interest included ‘any FA’ and the three most common types of FA: PA, egg allergy and milk allergy. As we reported previously, we adopted stringent clinical criteria to define a specific type of FA [35] : (1) a convincing history of clinical allergic reaction on ingestion of specific foods [35] and (2) evidence of sensitization to the same food, defined as having a detectable sIgE (≥0.10 kU l −1 ; detection limit of the instrument was <0.10 kU l −1 ) and/or a positive SPT to this specified food. A positive SPT for a specific allergen was defined based on criteria as follows: (1) the MWD for the negative control was <3 mm, the positive control was ≥3 mm and the difference of positive minus negative control was ≥3 mm; and (2) MWD was ≥3 mm for the specified allergen. Accordingly, we defined allergy to nine common foods (peanut, egg white, cow’s milk, soy, wheat, walnut, fish, shellfish and sesame seed) and ‘any FA’ if a child was allergic to any of these foods. Normal controls were defined if a child had neither clinical allergic reaction nor evidence of sensitization to any of the nine foods. All parents were defined as having uncertain FA phenotypes, as data on history of clinical allergic reaction subsequent to ingestion of specific foods were unavailable. We also performed sensitivity tests on FA definitions using other cutoffs for food-specific IgE and SPT, for example, food-specific IgE ≥0.35 kU l −1 , SPT MWD ≥5 mm (ref. 36 ) or either food-specific IgE or SPT MWD≥95% PPV. Genotyping and quality control steps in the discovery GWAS Genomic DNA was isolated from EDTA-treated peripheral white blood cells. The concentration and purity was determined using a Quant-iT Broad-range dsDNA Assay Kit on a SpectraMax M2 micro-plate reader. Genotyping was performed using the Illumina HumanOmni1-Quad BeadChip in the Genome Technology Access Center, Washington University in St Louis, MO, according to specifications listed in Illumina’s protocol (Illumina, Inc.). Among 2,759 genotyped samples, 12 failed to yield high-quality genotyping calls ( Supplementary Methods ), resulting in an overall genotyping success rate of 99.6%. Genotypes for 2,747 subjects were exported, with a total of 1,011,859 SNPs. We performed rigorous quality-control steps as suggested by Laurie et al . [59] , using the R/bioconductor package ‘GWASTools’ [60] . Briefly, we examined the following parameters: (1) missing call rate per SNP, per chromosome and per sample; (2) the reproducibility rate among the 100 duplicated samples; (3) duplicate discordance estimates for each SNP to infer SNP quality; 4) genotyping batch effects: measured by comparing the difference in allelic frequencies between each plate and a pool of the other plates, and by comparing variation in log 10 of the autosomal missing call rate in each plate (no significant batch effects were detected); (5) gender identity: based on X chromosome heterozygosity and the means of the intensities of SNP probes on the X and Y chromosome; (6) autosomal heterozygosity; (7) Hardy–Weinberg equilibrium (HWE) test: performed among self-reported Caucasian parents or a sibling without FA if no parent was available. Sex-specific HWE tests were also performed; (8) Mendelian error check of 650 families with both parents available; and (9) pair-wise sample relatedness: pair-wise kinship estimates between every subject were computed using PLINK [61] . We filtered 45,100 monomorphic SNPs and 14,948 SNPs with a >5% missing genotyping rate. A total of 595 SNPs with duplicate discordance estimates >2% in 98 pairs of duplicates and 1,784 SNPs that deviated from the HWE test ( P <1 × 10 −6 ) were also filtered. Mendelian error checks filtered 2,145 SNPs with Mendelian errors in ≥10 families (>1.5% families). Some SNPs were filtered under more than one criterion. We also removed 162,283 SNPs with minor allele frequency (MAF) <2% and 2,086 SNPs on the Y chromosome or on mitochondrial chromosomes. Finally, a total of 772,141 autosomal SNPs and 17,536 SNPs on the X chromosome were used in the downstream analyses. We removed one subject with a missing genotyping call rate >5%, 12 subjects with gender discrepancies and 6 subjects with Mendelian errors in >5,000 SNPs. Pair-wise relatedness was checked for each pair of subjects by plotting the proportion of loci where the pair shared one allele identical by descent versus the proportion of loci where the pair shared zero allele identical by descent. A total of 34 subjects for whom the degree of relatedness was inconsistent with self-reported relationship were then removed. In total, 2,694 subjects were available for downstream data analyses. Genetic ancestry was carefully computed by PCA using Eigenstrat [37] and all European, American, African and Asian individuals in the 1000 Genomes Project were used as a reference (phase I, release_v3.20101123), as detailed in Supplementary Methods . Statistical analyses in the discovery GWAS To leverage the family-based data with a small number of case–control samples, the MQLS test (for autosomal markers) [33] and its’ extension, the XM test [34] (for X-linked markers) were applied to explore genetic associations for each phenotype of interest using MQLS-XM ( http://www.stat.uchicago.edu/~mcpeek/software/MQLS_XM/download.html ), a programme for dichotomous outcomes. The MQLS can maximally use information available in a complex family structure by the following: (1) distinguishing between unaffected controls and controls of uncertain phenotypes (that is, individuals with unmeasured phenotypes), and incorporating both into the analyses; and (2) incorporating phenotype data for relatives with missing genotype data at each marker tested [33] . MQLS is a retrospective score test that treats the genotype data on sample individuals as random and the available phenotype information as fixed in the analysis, thus allowing for valid association testing in the presence of phenotype misspecification, and hence the method provides high power at the appropriate type I error rate [33] . Before the MQLS analysis, using PA as an example, the phenotype of interest was coded as follows: (1) PA-affected cases, (2) non-allergic non-sensitized normal controls and (3) controls of uncertain phenotypes (including children who did not meet the PA case or normal control definition, and all genotyped parents). We also performed a sensitivity test and found that the results were not significantly altered by removing children who did not meet the PA case or normal control definition from the analysis. The MQLS test was performed under an additive genetic model, with a specified prevalence of 5% for any FA or 1% for PA, milk allergy and egg allergy, separately, in the Europeans. We also repeated the analyses, while specifying a higher prevalence (10% for any FA, or 5% for PA, milk allergy and egg allergy, separately) and obtained very similar results. To perform MQLS analyses by conditioning on one of the top SNPs, we first calculated the residual using logit( Y =1)= β 0 + β G * G for subjects with non-missing phenotypes, where Y is the disease status and G is the genotype of the selected top SNP. The residual was set to 0 for subjects with missing phenotype. Similarly, to perform MQLS analyses in 497 non-European subjects adjusting for ancestry, the residual PA status for subjects with non-missing phenotypes was calculated using the first three PCs from the GWAS genotyping data as covariates and the residual for subjects with missing phenotypes was set to 0. The calculated residual was then used as the outcome to perform MQLS analyses using the QM-QXM programme, an approach that is an extension of the MQLS test to quantitative traits ( http://faculty.washington.edu/tathornt/software/QM_QXM/ ). As the MQLS is a score test and does not estimate effect size, the reported OR and 95% CIs were estimated using GEE models, with adjustment for age and gender in subjects of European ancestry. The first three PCs were also adjusted in the analyses for non-European subjects. Genotyping and data analyses in the replication sample The replication sample consisted of 88 PA cases and 128 normal controls from the same Chicago Food Allergy Study. SNPs rs7192 and rs9275596, which were suggestively or significantly associated with PA in the discovery GWAS ( P <1 × 10 −7 ), were selected for replication. As we needed to impute population ancestry using a similar strategy as was used for the discovery sample, and impute classical HLA alleles and AA polymorphisms based on a relatively dense SNP set, the Human OmniExpressExome BeadChip was selected for genotyping. DNA samples were prepared using the same lab procedures as for the discovery sample, and cases and controls were distributed evenly in each plate. Genotyping was performed according to specifications listed in Illumina’s protocol (Illumina, Inc.) at the Genomics Core Facility of the Department of Genetics and Genomic Sciences, Icahn School of Medicine at Mount Sinai. Similar quality-control steps were applied to the replication sample. Two subjects with gender inconsistencies and one subject from a monozygotic twin pair were removed from the subsequent data analysis. GEE models, adjusting for age and gender, were performed to test the association between each SNP and PA under an additive genetic model, in samples with European ancestry. When analyses were performed in samples of non-European ancestry, the first three PCs from the genome-wide SNP genotyping data were also included as covariates to adjust for potential population stratification. SNP imputation In the discovery sample, we performed phasing using SHAPEIT [38] and imputation using IMPUTE2 (ref. 39 ) with all individuals in the 1000 Genomes Project as a reference panel. As MQLS does not support analyses using posterior probabilities, we computed best-guess genotypes, using a probability threshold of 0.95, as recently described in the literature [62] . We applied several post-imputation quality-control metrics including removal of SNPs with an IMPUTE2 info score <0.8, with a missing call rate >0.05, or with a MAF <0.02. A total of 6,459,842 genotyped or imputed SNPs were then analysed for their associations with any FA and three specific types of FA, respectively, using the MQLS test. Meta-GWAS SNP imputation was also performed for the replication sample of European ancestry, leading to a combined set of 6,174,271 genotyped or imputed SNPs. We performed the association tests for PA in the replication sample using the GEE model (in a case–control setting), adjusting for age and gender, similar to what was done for genotyped SNPs rs7192 and rs9275596. To maximize power, we performed meta-analysis based on the Stouffer’s weighted z -score method to combine the association results for PA from the discovery and the replication samples. Our GEE analyses in the replication sample did not include SNPs on the X chromosome ( N =139,697) because of the small replication sample size and need to perform gender-specific GEE analyses (57 females and 74 males), and thus the meta-analysis was limited to 5,693,167 autosomal SNPs that overlapped in both sample sets. Imputation of HLA alleles and AA polymorphisms We used the HLA*IMP [41] programme to impute classical HLA alleles from SNP genotyping data via reference to a training data set of over 2,500 samples of European ancestry with dense SNP data and classical HLA allele types. This framework is reported to have high imputation accuracy (92%–98% of imputations agree with lab-derived HLA types) [41] . We also applied the SNP2HLA framework to impute AA polymorphisms as well as classical HLA alleles, with genotype data from the Major Histocompatibility Complex Working Group of the Type I Diabetes Genetics Consortium as a reference panel [42] . The imputation was performed for subjects of European ancestry in the MHC class II gene region. We used best-guess genotypes for analyses, as MQLS does not support analysis using posterior probabilities. After applying several quality-control filters to the imputed data (that is, removal of imputed variants with call rate <95% and/or MAF <0.02), 50 four-digit HLA alleles from the HLA*IMP programme, 27 two-digit HLA alleles, 41 four-digit alleles and 165 AA polymorphisms from the SNP2HLA programme were analysed for their associations with PA, using the MQLS test in the discovery sample and using the GEE model in the replication sample, as described above. Multiallelic AA polymorphisms were analysed for associations with PA after converting K-alleles to K-bialleles. DNA methylation measurement and quality-control steps A total of 218 unrelated children of European ancestry in the discovery ( N =199) or replication ( N =19) samples had genome-wide DNAm data measured in genomic DNA isolated from EDTA-treated peripheral white blood cells. DNAm was measured using Infinium HumanMethylation450 BeadChips (including >485,000 CpG sites), according to the manufacturer’s instructions at the Center for Genetic Medicine, Northwestern University Feinberg School of Medicine. Several quality-control steps were performed with the ‘minfi’ framework [63] , as detailed in the Supplementary Methods . Both β -and M -values (representing methylation ratios) were computed for downstream analyses. M -values are reported as superior to β -values for identification of differential methylation [64] . To account for potential batch effects, β - and M -values were ComBat-transformed using the ‘sva’ package [65] , with chip number as the surrogate for batches. The ComBat-transformed β - and M -values at each CpG site were applied to explore associations between DNAm, genotypes and PA. Cell heterogeneity in blood may act as a potential confounder [55] , [56] due to cell-specific patterns of DNAm [57] . Thus, with estimateCellCounts() function included in the ‘minfi’ package [63] , the distribution of six cell types (CD8T cells, CD4T cells, NK cells, B cells, monocytes and granulocytes) was inferred for each sample based on external reference DNAm signatures of the constituent cell type from Illumina HumanMethylation450 BeadChips [55] , [56] . The estimated cell composition was adjusted as a covariate in subsequent analyses. Statistical analyses on DNA methylation mediation effects To identify DMPs associated with the two validated PA-associated SNPs, we applied the ‘limma’ package [58] in R/bioconductor, to fit a linear regression model in 218 unrelated children of European ancestry, with ComBat-transformed M -values at each CpG site ( N =456,513) as a function of each SNP (under an additive genetic model), adjusted for age, gender and estimated cell composition. Genome-wide significance ( P <5 × 10 −8 ) cutoffs were applied. To report adjusted methylation differences in each genotype, ComBat-transformed β -values were analysed instead of ComBat-transformed M -values, which did not significantly change the results. The identified genotype-dependent DMPs were tested for associations with PA, by fitting a linear regression model with ComBat-transformed M -values as outcomes, adjusting for the covariates mentioned above. These analyses were conducted in 73 PA cases and 67 controls, while the remaining 78 children with uncertain PA phenotypes were removed from these analyses. Bonferroni correction was applied to adjust for multiple testing. To report adjusted methylation differences in each group, ComBat-transformed β -values were analysed instead of ComBat-transformed M -values, which did not significantly change the results. The SNP–DMP–PA relationships were then assessed using the CIT classification as methylation mediated, consequential, or independent [40] . We focused on the top DMP from each gene that was significantly associated with both SNPs and PA risk. Briefly, the CIT performs statistical tests for four conditions, all of which must be met to conclude that methylation mediation is occurring: (i) genotype and phenotype of interest (PA in the current study) are associated; (ii) genotype is associated with DMP after adjusting for phenotype; (iii) DMP is associated with phenotype after adjusting for genotype; and (iv) genotype is independent of phenotype after adjusting for DMP. The CIT P -value is defined using the intersection-union test framework as the maximum of the four-component test P -values. As the CIT was originally designed for continuous phenotypes, we applied a modified version based on logistic regression to examine the causal relationship for each SNP–DMP–PA pair in this study, which has been reported previously [32] . Functional annotation using existing eQTL data sets To identify potentially causal gene(s) underlying the identified genetic associations with PA, we queried existing eQTL databases in multiple tissues (including subcutaneous/omental adipose tissue [43] , liver tissue [43] and lymphocytes [44] , [45] , [46] ( http://regulome.stanford.edu )), to assess whether the top PA-associated SNPs were eQTL SNPs. We surveyed both cis - and trans -eQTLs of 10% false discovery rate and found that the two PA-associated SNPs influence gene expression mainly in a cis manner, and that corresponding cis -eQTLs were reported in the paper. For each gene whose expression level was significantly associated with the two PA-associated SNPs, the most significant cis -eQTL in the subcutaneous/omental adipose and liver tissues, separately, and its LD squared correlation coefficient with the PA-associated SNPs were also reported. How to cite this article: Hong, X. et al . Genome-wide association study identifies peanut allergy-specific loci and evidence of epigenetic mediation in U.S. Children. Nat. Commun. 6:6304 doi: 10.1038/ncomms7304 (2015).